Quasiparticles and Fermi liquid behaviour in an organic metal Many organic metals display exotic properties such as superconductivity, spin-charge separation and so on and have been described as quasi-one-dimensional Luttinger liquids. However, a genuine Fermi liquid behaviour with quasiparticles and Fermi surfaces have not been reported to date for any organic metal. Here, we report the experimental Fermi surface and band structure of an organic metal (BEDT-TTF) 3 Br( p BIB) obtained using angle-resolved photoelectron spectroscopy, and show its consistency with first-principles band structure calculations. Our results reveal a quasiparticle renormalization at low energy scales (effective mass m *=1.9 m e ) and ω 2 dependence of the imaginary part of the self energy, limited by a kink at ~50 meV arising from coupling to molecular vibrations. The study unambiguously proves that (BEDT-TTF) 3 Br( p BIB) is a quasi-2D organic Fermi liquid with a Fermi surface consistent with Shubnikov-de Haas results. Organic metals have an increasingly important role in safe and sustainable applications, ranging from stretchable electronics and photovoltaics to bio-integrated devices [1] , [2] . However, in spite of their discovery nearly 40 years ago [3] , it has not yet been possible to quantify the energy( ω ) and momentum( k )-resolved band dispersions and Fermi surfaces of any organic metal in terms of a genuine Fermi liquid [4] . In contrast, some organic metals possessing quasi-one-dimensional (1D) structure are classified as Luttinger liquids, with missing quasiparticles and a power-law density of states that forbid Fermi surface determination [5] , [6] , [7] , [8] . Quasi-2D metals bridge the Fermi–Luttinger paradigms and embody novel concepts such as marginal Fermi liquids [9] and spin-charge stripes [10] , but angle-integrated measurements for 2D organic metals have instead suggested Luttinger liquid character [11] , [12] , [13] . Organic materials indeed display a fascinating range of properties [14] , [15] , [16] including superconductivity, spin- and charge-density waves, photo-induced phase transitions, magnetism and so on. The electronic properties of these materials are derived from the electronic structure near the Fermi level ( E F ), but it is surprising that it has not yet been possible to describe the spectral function A( k , ω ) of any organic metal in terms of basic Fermi liquid behaviour. Angle-resolved photoelectron spectroscopy (ARPES) can directly provide the spectral function A( k , ω ) modulo matrix element effects [17] . However, ARPES studies of organic metals have been reported only for quasi-1D systems and indicate a Luttinger liquid picture in the absence of quasiparticles, as exemplified by studies on the Bechgaard salts [5] , TTF-TCNQ [6] , [7] , [8] and so on. (TTF, tetrathiafulvalene; TCNQ, 7,7,8,8-tetracyanoquinodimethane) Earlier attempts to measure A( k , ω ) of quasi-2D organic metals have not succeeded to measure quasiparticle bands dispersing across the Fermi level ( E F ). On the other hand, angle-integrated studies [11] , [12] , [13] of quasi-2D organic metals have always reported a power law dependence of the density of states, suggestive of Luttinger liquid behaviour like in the quasi-1D organic metals. For example, studies on (BEDT-TTF) 2 X salts (BEDT-TTF, bis(ethylenedithio)tetrathiafulvalene) reported absence of a Fermi edge and this was attributed to strong correlations [12] , [13] , whereas one study also discussed phonon excitations as a possible origin of the behaviour [11] . Most of the BEDT-TTF-based two-dimensional organic materials are 2:1 salts of the formula (BEDT-TTF) 2 X, with a structure of alternating BEDT-TTF and anion X layers [14] , [15] , [16] . The formal charge of BEDT-TTF is +1/2 in these systems and the conduction band is quarter-filled. If the structure results in a dimerization, as in the β- and κ-phase salts (with two dimers of BEDT-TTF molecules in a unit cell), the electron configuration leads to an 'effectively' half-filled strongly correlated electron system. These effects make organic materials very interesting and indeed, realizations include Mott insulators and superconductivity, as well as specific details such as pseudogap behaviour, a mid-infrared feature and electronic transport properties quite like the strongly correlated layered copper oxide superconductors [18] . Consequently, exotic phases can indeed be realized owing to choice of the anion, amount of band filling and the role of correlations, and extensive work has focused on the quasi-2D (BEDT-TTF) 2 X series of compounds [14] , [15] , [16] , [19] , [20] . Most importantly, Shubnikov-de Haas (SdH) quantum oscillations have identified a closed Fermi surface for some BEDT-TTF-based systems [21] . This indicates a contradiction because the angle-integrated photoemission spectroscopy (PES) studies concluded a Luttinger liquid behaviour in the absence of a Fermi edge [11] , [12] , [13] . In this work, we study the electronic structure of a quasi-2D compound (BEDT-TTF) 3 Br( p BIB) ( p BIB, p -bis(iodoethynyl)benzene), which can be considered to be a good metal in terms of electrical resistivity ρ ( T =4 K) ~100 μ Ωcm. The formal charge of the donor is not +1/2 but +1/3 and the crystal structure consists of the a , c lattice parameters being nearly equal ( a =10.187 Å, c =9.418 Å) and a substantially larger b lattice parameter ( b =15.420 Å). The crystal structure is shown in Fig. 1a and it satisfies a lattice matching between the BEDT-TTF layer and the infinite anionic chain made of p BIBs and bromide ions without a dimerization of the BEDT-TTF molecules. Electronic structure calculations indicate a quasi-2D behaviour [22] and indeed, a quasi-2D-closed Fermi surface has been confirmed by cyclotron resonance and SdH oscillations [21] , as well as angular-dependent magneto-resistance oscillations [23] , [24] at T =1.4 K. In the following, we present PES as well as ARPES studies of the electronic structure of (BEDT-TTF) 3 Br( p BIB). The experimental geometry is shown in Fig. 1b . Also, in spite of its large unit cell with a volume of 1,371.5 Å 3 , it was possible to carry out reliable first-principles band structure calculations. The ARPES results reveal band dispersions and the experimental Fermi surface, consistent with first-principles band structure calculations. The highest occupied molecular orbital (HOMO) electrons have S 3p character and undergo band renormalization consistent with SdH results. Laser ARPES results indicate Fermi liquid behaviour, with a kink at ~50 meV arising from coupling to molecular vibrations. 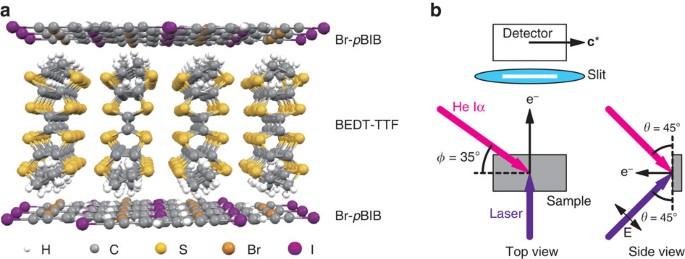Figure 1: Crystal structure and experimental geometry. (a) Crystal structure of (BEDT-TTF)3Br(pBIB). (b) Schematic diagram of experimental geometry showing the orientation of the incident Laser and He Iα sources with respect to the detector. The analyser slit is parallel toc*, wherec* is the reciprocal lattice vector ofcaxis of (BEDT-TTF)3Br(pBIB)22. Figure 1: Crystal structure and experimental geometry. ( a ) Crystal structure of (BEDT-TTF) 3 Br( p BIB). ( b ) Schematic diagram of experimental geometry showing the orientation of the incident Laser and He Iα sources with respect to the detector. The analyser slit is parallel to c *, where c * is the reciprocal lattice vector of c axis of (BEDT-TTF) 3 Br( p BIB) [22] . Full size image 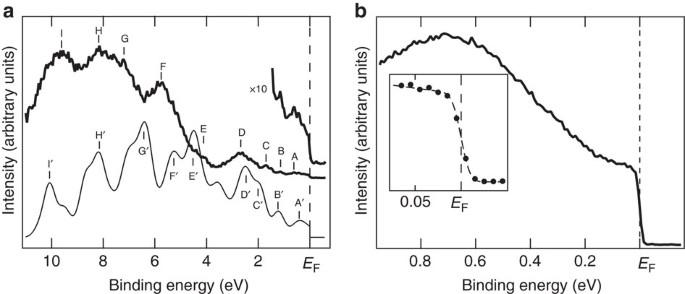Figure 2: Angle-integrated results and first-principles calculations. Angle-integrated photoemission spectra of (BEDT-TTF)3Br(pBIB) measured at 4 K using the photon source of (a) He Iα (bold line), plotted along with first-principles band structure calculations broadened by convolving with a Gaussian corresponding to the experimental energy resolution (thin line). Labels A–I and A′–I′ mark features in the experimental spectrum and first-principles band calculations, respectively. (b) The laser-PES data measured for (BEDT-TTF)3Br(pBIB) up to a binding energy of 1 eV below the Fermi level (solid line). Inset shows the spectrum nearEFindicating the existence of a metallic Fermi edge (circle), which can be well reproduced by a Fermi–Dirac function convolved with a Gaussian corresponding to the experimental energy resolution (broken line). Valence band measurements and first-principles calculations Figure 2a shows the wide-energy angle-integrated valence band spectrum of (BEDT-TTF) 3 Br( p BIB) obtained at 4 K using He Iα photons (21.218 eV) compared with the density of states obtained from first-principles band structure calculations. The features labelled A–I in the experimental spectra show a one–one correspondence with features A′–I′ in the calculated spectra, although small discrepancies can be seen in the features. The spectrum plotted on a magnified y -scale (×10) shows a clear Fermi edge. Figure 2b shows the near E F spectrum obtained at T =4 K using a laser source (6.994 eV) [25] and a high-energy resolution (14 meV), confirming a clear Fermi edge. The states at and near the Fermi level constituting the HOMO have S 3p character, as obtained from band structure calculations. As discussed in the introduction, a Fermi edge in a quasi-2D organic metal has not been observed in earlier studies. In the following, we investigate band dispersions and the Fermi surface responsible for the metallicity. Figure 2: Angle-integrated results and first-principles calculations. Angle-integrated photoemission spectra of (BEDT-TTF) 3 Br( p BIB) measured at 4 K using the photon source of ( a ) He Iα (bold line), plotted along with first-principles band structure calculations broadened by convolving with a Gaussian corresponding to the experimental energy resolution (thin line). Labels A–I and A′–I′ mark features in the experimental spectrum and first-principles band calculations, respectively. ( b ) The laser-PES data measured for (BEDT-TTF) 3 Br( p BIB) up to a binding energy of 1 eV below the Fermi level (solid line). Inset shows the spectrum near E F indicating the existence of a metallic Fermi edge (circle), which can be well reproduced by a Fermi–Dirac function convolved with a Gaussian corresponding to the experimental energy resolution (broken line). 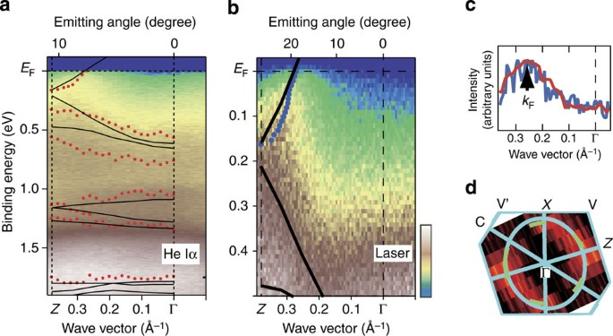Figure 3: Angle-resolved band map and Fermi surface. ARPES band dispersion map as a function of binding energy and momentum. Maps obtained using (a) He Iα and (b) Laser. The experimentally determined band dispersions are overlaid as symbols for He Iα (red circles) and for the laser (blue circles). Solid lines are the result of first-principles band calculations. (c) MDC atEFobtained from the He Iα ARPES map shown in panel (a), plotted as a red line, and from the laser-ARPES map of panel (b), plotted as a blue line. Both MDCs show the samekF, confirming quasi-2D behaviour (d) Fermi surface mapping using He Iα photon source. Light blue lines are the Brillouin zone and the Fermi surface calculated by a tight binding method22. Green broken line is the Fermi surface obtained from ARPES measurements. Full size image Angle-resolved band maps and Fermi surface Figure 3 shows ARPES spectra at 4 K along Γ–Z high-symmetry line using (a) He Iα and (b) laser photon source. The calculated band dispersions are overlaid as lines on the experimental band maps. The experimentally determined band dispersions are also overlaid as symbols for the He Iα measurements (red circles) and for the laser measurements (blue circles). Although the overall behaviour is quite consistent with the calculated band dispersions, small but finite deviations can be observed in the experimental band structure. However, the deviations do not depend on the photon energy and although the difference in incident photon energies is significantly large, the energy- and momentum-distribution curves (EDCs and MDCs) show very similar behaviour. Moreover, the E F crossing occurs at exactly the same Fermi momentum ( k F =0.27±0.005 Å −1 ) as seen from the MDCs at E F plotted in Fig. 3c . This also confirms that the electronic structure is quasi-2D and there is negligible dispersion perpendicular to the conducting ac -plane. From angle-dependent measurements using He Iα, we have mapped the Fermi surface in the a*c* -plane. The experimental Fermi surface is plotted in Fig. 3d along with the calculated Fermi surface [22] . While the calculated Fermi surface is elliptical, it is difficult to determine whether the experimental Fermi surface is elliptical or circular because of the low angular resolution perpendicular to Γ–Z direction. However, the observed Fermi surface crossing is consistent with SdH results [21] , [23] , [24] which indicated a circular Fermi surface with k F =0.27 Å −1 . The estimated cross-sectional area is 47% of the first Brillouin zone in ARPES, whereas it was estimated to be ~51% from the SdH results. Although inter- and intra-molecular band dispersions were recently reported for an insulating sexiphenyl film using ARPES [26] , the present result constitutes the only case of an experimentally measured k -resolved Fermi surface of an organic metal. Figure 3: Angle-resolved band map and Fermi surface. ARPES band dispersion map as a function of binding energy and momentum. Maps obtained using ( a ) He Iα and ( b ) Laser. The experimentally determined band dispersions are overlaid as symbols for He Iα (red circles) and for the laser (blue circles). Solid lines are the result of first-principles band calculations. ( c ) MDC at E F obtained from the He Iα ARPES map shown in panel ( a ), plotted as a red line, and from the laser-ARPES map of panel ( b ), plotted as a blue line. Both MDCs show the same k F , confirming quasi-2D behaviour ( d ) Fermi surface mapping using He Iα photon source. Light blue lines are the Brillouin zone and the Fermi surface calculated by a tight binding method [22] . Green broken line is the Fermi surface obtained from ARPES measurements. 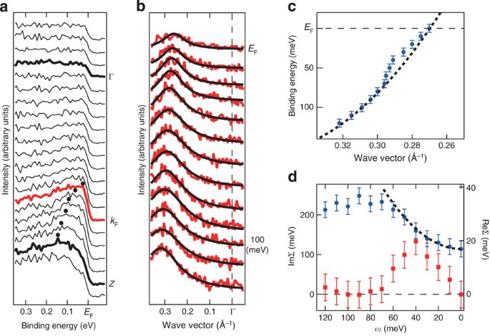Figure 4: Band dispersion and the self energy of quasiparticles. (a) Normalized EDCs obtained from the laser ARPES band map ofFig. 3bshowing a weak but definite quasiparticle band crossing (red curve). (b) MDCs obtained from the laser ARPES band map ofFig. 3b. Solid lines are the Lorentz function fits for each MDC. (c) Experimental band dispersion fromFig. 3b(blue circles) with the parabolic band (dashed line) assuming a free electron band. (d) Self-energy extracted from MDCs inFig. 4b. Results for ReΣ and ImΣ are shown as red squares and blue circles with experimental error bar, respectively. Dashed line indicatesω2behaviour, which well reproduces the ImΣ upto ~50 meV, corresponding to the kink energy observed in ReΣ as a peak. Full size image EDCs, MDCs and self energy of quasiparticles Figure 4a,b shows the EDCs and MDCs obtained from the laser ARPES band map of Fig. 3b , respectively. While the EDCs do not show a clear dispersive quasiparticle peak, the MDCs show a clear peak structure as a function of momentum. From a careful comparison of the experimental data with a parabolic band ( Fig. 4c ), we could identify a weak kink structure and were able to quantify the real (Re) and imaginary (Im) parts of the self energy (Σ). The results of such an analysis are shown in Fig. 4d . The Re Σ shows a peak structure centred at 40~50 meV associated with the kink structure observed in Fig. 4c . In addition, the Im Σ shows a clear ω 2 dependence (dotted line). It is noted that the ω 2 dependence is theoretically well known for a 3D metal with electron–electron correlations, whereas for a 2D metal with electron–electron correlations, the expected behaviour is Im Σ ω 2 {1+ β ln( ω / E F )} and for a 2D electron–phonon coupled system it is known to show an ω 2 dependence due to many body effects [27] . As our ARPES studies as well as earlier SdH results indicate a quasi 2D electronic structure, we need to address the importance of electron–phonon coupling in (BEDT-TTF) 3 Br( p BIB). To do so, we note that the ω 2 dependence occurs up to an energy scale of the kink structure. The kink structure arises from coupling of electrons to a bosonic mode, which could be phononic, magnetic and so on [17] . We could estimate the electron–boson dimensionless coupling parameter λ =0.9 from the experimental data using standard procedures [17] . The estimated effective mass for the carriers is m *=1.9 m e , whereas the SdH results indicated an effective mass ( m *=2.0 m e ), indicating very good agreement between the two techniques. Figure 4: Band dispersion and the self energy of quasiparticles. ( a ) Normalized EDCs obtained from the laser ARPES band map of Fig. 3b showing a weak but definite quasiparticle band crossing (red curve). ( b ) MDCs obtained from the laser ARPES band map of Fig. 3b . Solid lines are the Lorentz function fits for each MDC. ( c ) Experimental band dispersion from Fig. 3b (blue circles) with the parabolic band (dashed line) assuming a free electron band. ( d ) Self-energy extracted from MDCs in Fig. 4b . Results for ReΣ and ImΣ are shown as red squares and blue circles with experimental error bar, respectively. Dashed line indicates ω 2 behaviour, which well reproduces the ImΣ upto ~50 meV, corresponding to the kink energy observed in ReΣ as a peak. Full size image In the absence of experimental studies of phonons in (BEDT-TTF) 3 Br( p BIB), we have compared with molecular vibration modes known from optical spectroscopy of superconducting (BEDT-TTF) 2 Cu(NCS) 2 . Such a comparison helps to quantify the electron–phonon coupling strength of molecular vibration modes in (BEDT-TTF) 3 Br( p BIB) in relation to superconducting (BEDT-TTF) 2 Cu(NCS) 2 . The optical spectra of (BEDT-TTF) 2 Cu(NCS) 2 reported earlier was analysed on the basis of neutral BEDT-TTF molecules [28] . The spectra of (BEDT-TTF) 2 Cu(NCS) 2 indicated several modes with main features at about 20, 40, 60, 112 meV and a doublet at 182 and 187 meV. Using a simplified tight-binding analysis for the HOMO electrons and their coupling to the vibrational modes of the BEDT-TTF molecule, an electron–phonon coupling parameter of λ ph =0.37–0.45 was estimated [29] . The results also showed that the electron–phonon coupling is the strongest for the ~60-meV mode and it does not change across the superconducting transition. Thus, the presently obtained value of λ =0.9 from ARPES studies is about twice the value estimated from optical studies of BEDT-TTF-based organic superconductors. This indicates that the intra-molecule vibrations couple quite strongly to the carriers forming the Fermi surface and have an important role in the electronic structure of (BEDT-TTF) 3 Br( p BIB) also. Based on the above characteristics and the fact that the kink energy matches with low-energy vibration mode known from optical studies, we attribute the kink feature observed in our ARPES data to electron–phonon coupling, although we cannot definitively rule out the role of electron–electron correlations in 2D. From the E F band crossing, the Fermi velocity is estimated to be v F =2.0 eVÅ. This indicates a relatively high Fermi velocity renormalized metal for (BEDT-TTF) 3 Br( p BIB) belonging to the BEDT-TTF family of exotic metals. Synthesis and the crystal structure High-quality single crystals of (BEDT-TTF) 3 Br( p BIB) were grown by electrochemical oxidation of BEDT-TTF in the presence of tetraphenylphosphonium bromide and p BIB dissolved in chlorobenzene (5% MeOH) [22] . The crystal structure data were measured under the same conditions of cooling rate and temperature as for the ARPES measurements so as to ensure a reliable comparison between experimental results and the first-principles band calculations. First-principles band calculation The calculation method and details are basically the same as those reported in ref. 30 . The calculations are based on the density functional theory within the generalized gradient approximation. The experimentally determined low-temperature crystal structure was used for the first-principles band structure calculations. Planewave basis sets are used with the ultrasoft pseudopotential technique. The cutoff energy for wave functions is 25 Ry and 256 Ry for charge density. ARPES experiment The He Iα ARPES measurements were performed on a spectrometer built using a hemispherical electron analyser (GAMMADATA-SCIENTA SES2002) and a high-flux He discharge lamp with a toroidal grating monochromator, which gives partially polarized photons. The schematic of the spectrometer geometry is shown in Fig. 1b . Although the geometry allows symmetry-selective polarization-dependent ARPES using laser source, the geometry is not suitable for symmetry-selective ARPES using the He discharge lamp. The spectra were measured with He Iα resonance line (21.218 eV) at a vacuum of ~1×10 −10 Torr during measurements and a base vacuum of <5×10 −11 Torr. The laser-ARPES measurements were carried out using a hemispherical electron analyser (VG-SCIENTA R4000) and a quasi-continuous wave narrowband ultraviolet laser (6.994 eV), with an operating vacuum of ~5×10 −11 Torr during measurements and a base vacuum of <2×10 −11 Torr. The total energy resolution (analyser and light) was set to 36±2 meV for He Iα measurements and 14±2 meV for laser measurements. The angular resolution was set to 0.33° corresponding to k resolution of ±0.012 Å −1 for He Iα measurements and 0.36° corresponding to k resolution of ±0.0052 Å −1 for laser measurements. Samples were mounted on an original-designed double-walled gold-plated thermally shielded sample holder, and the sample temperature was measured using a calibrated silicon diode sensor mounted just below the sample, with an accuracy of ±0.1 K. Normalization of spectra was done with scan time. All the spectra reported here were measured on clean surfaces obtained by fresh in situ cleaves on the same sample, or for samples from the same batch. The samples were cleaved in situ at 4 K and resulted in flat, shiny metallic surfaces. The sample orientation was determined using X-ray diffraction and confirmed by the symmetry of the measured ARPES spectra. We have confirmed the absence of degradation effects and highly reproducible spectra over a period of 3 h after cleaving. The reproducibility of the ARPES spectra was established by repeated measurements on freshly cleaved surfaces. Also, the reproducibility of the He Iα and laser-ARPES measurements for the Fermi surface crossing shows that the surface sensitivity is not a problem and the obtained spectra represent the intrinsic electronic structure of (BEDT-TTF) 3 Br( p BIB). The Fermi edge ( E F ) of samples was referenced to that of a gold film evaporated onto the sample substrate. The total energy resolution is determined by fitting the E F spectrum of (BEDT-TTF) 3 Br( p BIB) to the Fermi–Dirac distribution function at 4 K convolved with a Gaussian. The accuracy in position of E F is ±1–2 meV. Self-energy analysis The self energy Σ was obtained using the method described in ref. 17 , which uses a spectral function of the form A( k , ω ) ImΣ( ω )/([ ω − −ReΣ( ω )] 2 +[ImΣ( ω )] 2 ), where is the non-interacting bare dispersion. ReΣ(ω) and ImΣ(ω) are directly extracted from MDCs. MDC fits were carried out using Lorentz functions and a least-squares method. For the bare dispersion, we have used a parabolic band instead of the calculated band dispersion result. However, we ensured that the parabolic band reproduces the experimental k F as well as the band dispersion at binding energies higher than the kink structure. ImΣ( ω ) are calculated from multiplying MDC width and bare band velocity. How to cite this article: Kiss, T. et al . Quasiparticles and Fermi liquid behaviour in an organic metal. Nat. Commun. 3:1089 doi: 10.1038/ncomms2079 (2012).